Metallized DNA nanolithography for encoding and transferring spatial information for graphene patterning The vision for graphene and other two-dimensional electronics is the direct production of nanoelectronic circuits and barrier materials from a single precursor sheet. DNA origami and single-stranded tiles are powerful methods to encode complex shapes within a DNA sequence, but their translation to patterning other nanomaterials has been limited. Here we develop a metallized DNA nanolithography that allows transfer of spatial information to pattern two-dimensional nanomaterials capable of plasma etching. Width, orientation and curvature can be programmed by specific sequence design and transferred, as we demonstrate for graphene. Spatial resolution is limited by distortion of the DNA template upon Au metallization and subsequent etching. The metallized DNA mask allows for plasmonic enhanced Raman spectroscopy of the underlying graphene, providing information on defects, doping and lattice symmetry. This DNA nanolithography enables wafer-scale patterning of two-dimensional electronic materials to create diverse circuit elements, including nanorings, three- and four-membered nanojunctions, and extended nanoribbons. Two-dimensional (2D) electronic materials such as graphene, a monolayer of sp 2 -bonded carbon atoms, are emerging as promising candidates for next-generation nanoelectronics [1] , [2] . An important vision for these materials is to enable complex and diverse circuit designs directly patterned from an initial monolayer [3] , [4] , [5] , thereby circumventing key challenges in the placement, orientation and electronic control of constituent nanocomponents, such as carbon nanotubes. In the case of graphene, nanopatterning can enable a diversity of electronic functions including quantum confined electronic band gaps in graphene nanoribbons [6] , [7] , quantum interference effects and Aharonov–Bohm oscillations in graphene nanorings [8] , [9] and single-electron transport in graphene quantum dots [10] , [11] . Previously demonstrated methods for forming graphene nanostructures and nanoribbons in the literature can be grouped into three main categories: (a) top-down etching methods based on larger graphene sheets [12] , [13] , (b) bottom-up synthesis methods from molecular building blocks [14] and (c) unzipping methods based on carbon nanotubes to form nanoribbons [15] , [16] . However, the preparative synthesis of arbitrarily shaped graphene nanostructures with specific spatial dimensions remains a significant challenge. For example, electron beam lithography (EBL) can be used for patterning graphene into specific shapes using a rastering approach, but cannot efficiently yield wafer-scale, pre-programmed graphene structures with sub-100 nm size. DNA self-assembly [17] , [18] , [19] , [20] , [21] , [22] , [23] , [24] , [25] , [26] , [27] , [28] , such as DNA origami [22] , [23] , [24] and single-stranded tile (SST) assembly [26] , [27] , [28] , can create complex 2D [22] , [24] , [26] , [27] and 3D [18] , [20] , [23] , [28] structures by encoding structural information using oligonucleotide recognition. Both the SST strategy—assembling a structure from hundreds of synthetic SSTs (most are 42-bases long)—and the DNA origami strategy—assembling a structure by folding a long single-stranded DNA scaffold (7–8-kb long M13 viral genome) via its hybridization with hundreds of short synthetic ‘staple strands’—permit the programming of complex 2D and 3D shapes with nanometre scale features. DNA nanostructures can be used to expand the morphological and functional diversity of other nanomaterials. For example, DNA nanostructures can template the positioning of nanoparticles and carbon nanotubes [29] , [30] , [31] , [32] , [33] and they can also be functionalized into metallic nanostructures [34] , [35] , [36] , [37] , [38] , [39] , [40] . However, the transfer of spatial information to other 2D materials remains unexplored. Metallization produces nanowires and particles composed of disconnected grains, which decrease the conductivity [34] , [35] , [36] , [37] , [38] , [39] , [40] . In this way, DNA metallization is limited in its ability to construct nanoelectronic devices [40] . DNA nanostructures have also been used as shadow masks for metal deposition [41] and SiO 2 etching [42] , [43] , [44] . However, unprotected DNA masks degrade under plasma exposure, hindering their use for nanolithography. For successful shape-specific lithography, the encoded information must be transferred to a more stable lithographic mask. Metallized DNA lithography Herein we demonstrate an important advance towards complex nanopatterning of graphene by employing metallized DNA nanostructures as lithographic masks. Single-stranded DNA molecules are encoded with structural information ( Fig. 1a ) and hybridized with their complementary partners at specific locations which causes them to assemble into the prescribed 2D planar shape in solution ( Fig. 1b ). The DNA template is then adsorbed onto the graphene surface with the aid of a 1-pyrenemethylamine adhesion layer ( Fig. 1c ). The DNA nanostructures are treated with glutaraldehyde to enable seeding with Ag [36] , and are subsequently coated with Au (see the Methods section). This metallization of the DNA template renders it into a lithographic gold mask on the graphene that largely preserves its original spatial information ( Fig. 1d ). The metallization allows the DNA template to survive the subsequent etching process and to function as a positive relief mask. Ar/O 2 plasma reactive ion etching (RIE) removes the unprotected region of graphene ( Fig. 1e ) while allowing transfer of the spatial information from the metallized DNA templates to the final etched graphene products after metal dissolution ( Fig. 1f ). 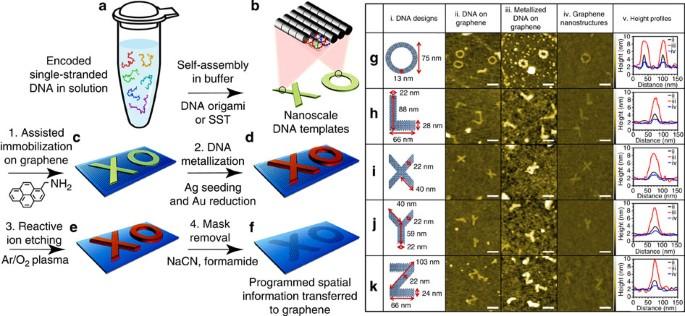Figure 1: Nanopatterning of graphene via metallized DNA structures that encode and transfer spatial information. (a) The encoded single-stranded DNA building blocks were programmed to fold into complex nanoscale DNA templates in solution. (b) Specific DNA templates, that is, X- and ring-shapes, were formed by DNA origami or SST. (c) Nano-sized DNA templates with specific shapes were deposited onto pre-synthesized graphene sheets (lithography step 1). (d) Metallization of the DNA templates generated custom-shaped gold masks on graphene (lithography step 2). (e) RIE removed unprotected graphene, leaving only gold mask-covered regions on wafer (lithography step 3). (f) Specifically shaped graphene nanostructures, that is, graphene X-shapes and nanorings, were obtained after mask removal (lithography step 4). (g–k) Graphene nanorings and letter-shapes derived from metallized DNA templates, from top to bottom, ring-, L-, X-, Y- and Z-shaped nanostructures, respectively. Columns (i–v), from left to right: (i) motif designs of DNA templates, (ii) AFM images of the DNA templates immobilized on graphene, (iii) the metallized templates on graphene, (iv) the final etched graphene shapes and (v) typical height profiles of the structures in column ii (black), iii (red) and iv (blue). Scale bars, 100 nm (AFM lateral); 10 nm (height scales). Figure 1: Nanopatterning of graphene via metallized DNA structures that encode and transfer spatial information. ( a ) The encoded single-stranded DNA building blocks were programmed to fold into complex nanoscale DNA templates in solution. ( b ) Specific DNA templates, that is, X- and ring-shapes, were formed by DNA origami or SST. ( c ) Nano-sized DNA templates with specific shapes were deposited onto pre-synthesized graphene sheets (lithography step 1). ( d ) Metallization of the DNA templates generated custom-shaped gold masks on graphene (lithography step 2). ( e ) RIE removed unprotected graphene, leaving only gold mask-covered regions on wafer (lithography step 3). ( f ) Specifically shaped graphene nanostructures, that is, graphene X-shapes and nanorings, were obtained after mask removal (lithography step 4). ( g–k ) Graphene nanorings and letter-shapes derived from metallized DNA templates, from top to bottom, ring-, L-, X-, Y- and Z-shaped nanostructures, respectively. Columns (i–v), from left to right: (i) motif designs of DNA templates, (ii) AFM images of the DNA templates immobilized on graphene, (iii) the metallized templates on graphene, (iv) the final etched graphene shapes and ( v ) typical height profiles of the structures in column ii (black), iii (red) and iv (blue). Scale bars, 100 nm (AFM lateral); 10 nm (height scales). Full size image We examined six types of DNA templates to test the transfer and preservation of spatial information (such angles and curvature) from the original DNA templates to eventual graphene nanostructures. A circular ring was designed using 3D DNA origami [24] , whereas various ‘letter-shaped’ junctions and a nanoribbon were designed using 1D and 2D SST [26] , [27] . Crude products for DNA nanorings and letter-shapes were purified by 2% native agarose gel electrophoresis. Monolayer graphene sheets were grown on copper foils via chemical vapour deposition (CVD) [45] and subsequently transferred to SiO 2 /Si wafers (300-nm thick SiO 2 layer) with the assistance of spin-coated poly (methyl methacrylate) (PMMA) films and a CuCl 2 /HCl copper etchant. The hydrophobic nature of CVD graphene hinders an evenly distributed deposition of the DNA nanostructures onto the CVD-graphene sheet. We found that pre-adsorption of 1-pyrenemethylamine molecules onto the graphene significantly increased the surface adhesion and improved the dispersion of negatively charged hydrophilic DNA templates on graphene, without damaging either the DNA structures or the underlying graphene (as demonstrated below by Raman measurements). We also tested cationic surfactants, such as cetrimonium bromide (CTAB) and sodium dodecyl sulfate (SDS), to improve the surface wetting of graphene towards the negatively charged DNA templates. However, we found that DNA nanostructures did not survive in the presence of such ionic surfactants. In control experiments, mask removal of metallized DNA on graphene by sequential soaking in NaCN and formamide without subsequent etching recovered intact graphene without residue or observable defects. Further experimental details can be found in the Methods section. The programming and transfer of DNA patterns is firstly demonstrated by the achievement of sub-100 nm graphene nanorings ( Fig. 1g ) that copied curvature from DNA templates. We also examined letter-shaped junctions, that is, L, X, Y and Z ( Fig. 1h–k ). The L-shaped DNA mask demonstrated the perpendicular alignment of two ribbons with different widths ( Fig. 1h ). The X-, Y-, and Z-shaped masks were used to demonstrate successful printing of junctions composed of two or three ribbons with distinct orientations ( Fig. 1i–k ). After each processing step, the morphological changes of deposited DNA templates, metallized DNA masks and final graphene nanostructures were investigated by atomic force microscopy (AFM) ( Fig. 1 h–k , column ii–v; also see Supplementary Table S1 for statistical analysis). The graphene nanostructures were produced at preparative scale and depending on the concentration of initial DNA templates deposited on graphene, several letter-shaped graphene patterns can be observed in an area of 1 μm 2 ( Fig. 1h–k , column iv). We note that the resolution of the lateral features under AFM scanning is limited by the sharpness of the AFM tip. The designed width of the DNA nanorings is 13 nm with a 75-nm outer diameter. The measured height and width of glutaraldehyde-treated DNA nanorings deposited on graphene are 2.9±0.3 and 16.1±1.3 nm, respectively. The small increase in the width of the DNA templates compared with their design is likely due to the partial dehydration and flattening of the soft DNA structures on the dry surface. After metallization, the height and width of DNA nanorings were measured as 7.2±1.4 and 29.4±3.2 nm, respectively, confirming the success of the Au reduction. The metallized DNA masks are composed of fused gold nanoparticles that nucleated along the DNA skeletons and induced the size expansion. Upon subsequent RIE etching and mask-removal processing, the final graphene nanostructures were obtained, with a height and width of 1.2±0.3 and 19.0±4.3 nm, respectively. Plasma beam scattering at the edges of mask during the RIE process appears to shrink the resulting graphene edges, producing a narrower structure than that of the metallized DNA mask. However, the ring structure was preserved throughout all steps of the nanolithography. The competing effects of size expansion by metallization and shrinking by the etching process result in the fairly accurate preservation of spatial information. The average outer diameter of the initial DNA masks and the final graphene nanorings were 75.7±5.6 and 81.7±5.4 nm, respectively, indicating successful transfer of this spatial feature. Similar fidelity was observed for the samples with letter-shaped DNA templates. The initial letter-shaped DNA templates deposited on graphene almost all have the same height, with an average value of 2.1±0.3 nm. The metallized DNA masks of letter-shapes showed a height distribution of 6.7±0.9 nm and an average arm-width increase from 20.9±2.9 to 31.4±5.0 nm. The final graphene nanostructures derived from all letter-shape templates has an average height of 1.1±0.2 nm, and the distribution of arm-width has fallen back to a lower value, which is slightly wider but still close to the width of initial DNA templates. The features of letter-shaped junctions were also well preserved after DNA nanolithography. The right angle of L-shaped graphene was determined to be 94.4±4.2°, in accordance with the right-angle value of 93.3°±1.8° measured from deposited L-shaped DNA template on graphene. We also examined the feature change in X-shaped samples; the X-shaped DNA templates had an average acute arm-angle of 72.9±5.0° and an average arm-length of 37.4±3.8 nm. After lithography steps, the resultant X-shaped graphene nanostructures showed an acute arm-angle of 75.0±6.4° and arm-length of 38.6±6.9 nm, which suggests that the symmetry of X-shaped junctions has remained intact. Similarly, the obtuse arm-angle of Y-shaped patterns has been changed from 141.1±14.4° in initial Y-shaped DNA template to 139.9±16.2° in Y-shaped graphene nanostructures. We found that the background deposition of metal nanoparticles on the substrate ( Fig. 1g–k , column iii) did not disrupt the graphene patterning, although some tiny graphene quantum dots derived from the dispersed metal nanoparticles were found after plasma etching and mask removal ( Fig. 1g–k , column iv). Generally, the shapes of the resulting graphene letter-shapes were well replicated from the original DNA templates, with the exception of a systematic increase in feature sizes and edge roughness inherited from the metallized DNA masks. The observed tolerances suggest that improvements in plasma beam scattering, and precision in the metallization step could allow for sub-10 nm widths. Compared with traditional approaches, such as EBL, using DNA nanostructures as templates to achieve diverse shaped conductive materials has some key advantages: mass production of distinct structures and relatively high fabrication resolution. Especially, the ring-shaped graphene nanostructures produced by DNA-templated lithography, with ~40 nm inner diameter and ~20 nm width, cannot be easily reproduced using EBL. Moreover, because this is the first pattern transfer from a DNA nanostructure to a conductive 2D material that we are aware of, we suggest this DNA nanolithography is an advance for the field and a promising application of the DNA self-assembly technology. Modelling the transfer of spatial information A central issue in this work is the transfer and partial degradation of spatial information from the DNA template to the final graphene structure after each step of the lithography (DNA template deposition, metallization, etching and mask removal). The boundary of the template surface T ( r ) imprinted in final form on the graphene can be represented as a probability distribution function, p [ T ], expressed as a convolution of T with transfer functions σ ( r ) that represent the distortion of spatial information in the each step of the lithography: Each lithography step preserves or distorts the emerging boundary through a series of transfer functions based on physical processes such that σ ( r )= σ 0 ( r )* σ 1 ( r )* σ 2 ( r )* σ 3,4 ( r ), where σ 0 ( r ) is the original spatial information programmed in the DNA template. For example, the shape-distortion processes corresponding to dry transfer to the graphene surface (lithography step 1), metallization (lithography step 2), and etching and mask removal (lithography step 3 and 4) approximate a Gaussian process σ i ( r )=exp(−( r − R ) 2 /4 D r, i t i ) after time t . Here, the effective diffusivity of step i, D r, i can be estimated from the actual experimental variances, as detailed in the Supplementary Table S1 . As a programmable template, DNA is unique in the spatial precision that it affords in transferring desired coordinates to the physical structure, approximating a delta function: σ 0 ( r )~ δ ( r − R ) for the boundary at R ( Fig. 2a ). Transfer to the dry substrate ( Fig. 2b ) distorts the template by compressing the height and altering the lateral dimensions through van der Waals contraction. However, the largest degradation of spatial information occurs during metallization, which involves two consecutive steps that reduce resolution: Ag seeding, which extends the surface boundary by the diameter of the nucleated particles, and Au deposition, which extends the already roughened boundary ( Fig. 2c ). Imperfections formed during the metallization step are clearly transmitted to the underlying graphene, and include irregularities in the mask width, and discontinuities in the mask edge at the junctions between Au nanoparticles. For example, C-shaped graphene or graphene arcs (see Supplementary Fig. S1 ), were occasionally observed besides graphene nanorings as byproducts, with breaks in the ring structure observed in addition to the average width distribution of 19.3±4.2 nm. The final etching and mask-removal step ( Fig. 2d ) is relatively non-dispersive but does contract the boundary in the radial direction as the plasma beam scattering in the lateral dimensions. From the convolution model, for the first time we show that spatial information is lost in very specific ways with each patterning step according to the physics and chemistry of the lithography process. For example, the metallization step has the disadvantage that it currently causes the dispersion of the boundary. One consequence of the model is its prediction that non-dispersive transfer steps are essential to precision in spatial patterning using this approach. In theory, if all the lithography steps could be replaced with those possessing minimal dispersion, information transfer from templates to nanopatterns could be perfect. Future work will explore other different patterning strategies that utilize the high fidelity of the DNA templates directly, hence enabling higher resolution. 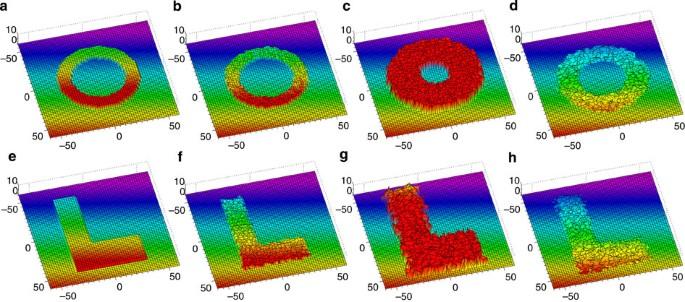Figure 2: Modelling the transfer of spatial information from the DNA templates to final graphene nanostructures. (a,e) The boundary of the original DNA templates programmed with specific shapes (ring- and L-shape). (b,f) The transfer of DNA templates to the dry substrate (lithography step 1) distorts the dimensions due to environmental interactions, such as the partial dehydration and flattening of soft DNA structures. (c,g) The metallization on DNA template (lithography step 2) expands its size and increased the roughness of boundary. (d,h) The RIE etching and mask removal (lithography step 3 and 4) shrinks the dimensions of final graphene nanostructures as the plasma beam scattering in the lateral edges. The unit of length scale in all images is nm, and the height and distance of the modelled nanostructures and substrate surface are indicated by the colour gradients. Figure 2: Modelling the transfer of spatial information from the DNA templates to final graphene nanostructures. ( a , e ) The boundary of the original DNA templates programmed with specific shapes (ring- and L-shape). ( b , f ) The transfer of DNA templates to the dry substrate (lithography step 1) distorts the dimensions due to environmental interactions, such as the partial dehydration and flattening of soft DNA structures. ( c , g ) The metallization on DNA template (lithography step 2) expands its size and increased the roughness of boundary. ( d , h ) The RIE etching and mask removal (lithography step 3 and 4) shrinks the dimensions of final graphene nanostructures as the plasma beam scattering in the lateral edges. The unit of length scale in all images is nm, and the height and distance of the modelled nanostructures and substrate surface are indicated by the colour gradients. Full size image Raman spectra and surface-plasmon enhancement We used Raman spectroscopy with an excitation wavelength of 633 nm to study the electronic and structural changes [46] , [47] , [48] , [49] that occur in the graphene during the different steps of the nanolithography. Typical Raman spectra ( Fig. 3a–d ) and deconvoluted G band structures ( Fig. 3e–h ) were collected after each lithography step over a ~1-μm spot size containing just one graphene nanostructure. All the Raman peaks were fit to Lorentzians after background subtraction for further analysis. Statistical information was collected for the integrated D band intensity, G band position, full width at half maximum (FWHM) of the 2D band and the intensity ratio of 2D and G bands ( I 2D / I G ), shown in Fig. 3i–l and additionally in Supplementary Table S2 . We observed that the shape of the DNA letter template (O-, X-, Y-, Z- or L-shape) does not influence the resulting Raman spectra because of their similar sizes; there is minimal variation in the Raman signal of the graphene patterns derived from the five different DNA letter-shapes for each lithography step. Therefore, the following analysis of Raman spectroscopy is based on the statistical results of all letter-shapes combined and is thus representative for each shape. 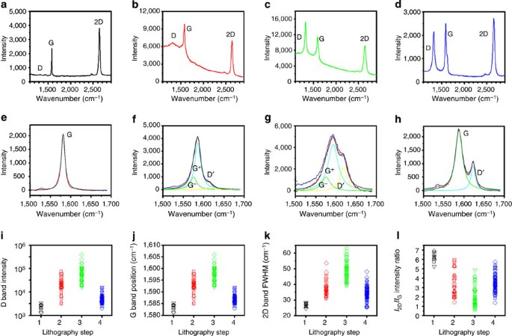Figure 3: Raman characterizations. Typical Raman spectra and the deconvolution of G bands of (a,e) graphene sheets with aforementioned DNA templates (lithography step 1), (b,f) graphene sheets with metallized DNA masks (lithography step 2), (c,g) after RIE etching (lithography step 3) and (d,h) graphene nanostructures after mask removal (lithography step 4). The overall statistical histograms of (i) integrated D band intensity, (j) G band position, (k) 2D band FWHM value and (l)I2D/IGvalue distribution of Raman spectra collected after each lithography step 1–4. Figure 3: Raman characterizations. Typical Raman spectra and the deconvolution of G bands of ( a , e ) graphene sheets with aforementioned DNA templates (lithography step 1), ( b , f ) graphene sheets with metallized DNA masks (lithography step 2), ( c , g ) after RIE etching (lithography step 3) and ( d , h ) graphene nanostructures after mask removal (lithography step 4). The overall statistical histograms of ( i ) integrated D band intensity, ( j ) G band position, ( k ) 2D band FWHM value and ( l ) I 2D / I G value distribution of Raman spectra collected after each lithography step 1–4. Full size image After deposition of the DNA template, the Raman spectrum ( Fig. 3a ) showed a minuscule D band, a G band at ~1,583 cm −1 and a sharp and single 2D band at ~2,638 cm −1 with a FWHM of <30 cm −1 , similar to pristine, largely defect-free graphene [47] . After metallization, the Raman spectrum ( Fig. 3b ) showed significantly increased scattering intensity, consistent with surface-enhanced Raman scattering (SERS) generated from the light-excited surface plasmons on gold nanostructures attached to the DNA template [50] . The average intensity of D, G and 2D bands increased by a factor of 9.6, 4.0 and 2.0, respectively. We observe that compared with the 2D band, the G band has a larger enhancement of the scattering cross-section, which is reflected in the decrease of the I 2D / I G value from 6.2 to 3.6. This is consistent with literature observations [50] , [51] , [52] and ascribed to a combination of doping-induced electron–phonon and electron–electron scattering [53] generated by the metal nanoparticles on metallized DNA masks as dopants [50] , [51] , [52] . A larger D band and a new D′ band at ~1,620 cm −1 appeared in the SERS spectra ( Fig. 3b ). The height increase of D band is assigned to the SERS enhancement, because the metallization process itself is not symmetry breaking and does not greatly increase the concentration of lattice defect sites on graphene sheets [51] . The Au metal deposition also dopes the graphene, as evidenced by the increase of the G peak position, the G and 2D peak width and decrease of the I 2D / I G value (lithography step 3 in Fig. 3i–l ) [47] . The splitting of the G band ( Fig. 3f ) into components at 1,580 cm −1 (G − ) and 1,592 cm −1 (G + ) is indicative of strained graphene [54] . The increase in the FWHM of 2D band (from 20 cm −1 after lithography step 1 to 37 cm −1 after lithography step 2) is an inhomogeneous broadening due to increased charge fluctuations in the graphene caused by different types of charge carriers [55] . An advantage of the nanolithography is that after RIE etching of the graphene, the remaining metallized mask generates a persistent SERS enhancement, allowing a sensitive assessment of symmetry breaking defects after the harshest step. Figure 3c show that the SERS persists and that there is a further up-shift of the G band to 1,597 cm −1 and of 2D band to 2,658 cm −1 , with a 49 cm −1 FWHM of 2D band. The I 2D / I G value further decreased to a value of 2.4. These changes are consistent with further doping. We also observed symmetry breaking by RIE etching as demonstrated by the strongly increased D and D′ band intensity with factors of 5.3 and 3.0, respectively. After the final mask removal ( Fig. 3d ), the SERS effect was eliminated as expected, yet strong D and D′ bands remain, consistent with permanent symmetry breaking from the patterning itself. Overall, the intensity ratio of D and G bands ( I D / I G ) approaches ~1.0 after mask removal; the D band is caused both by rough edges and the residual defects on the graphene structures [56] , [57] . The FWHM of G and 2D bands were greatly decreased after mask removal, with a downshifting back to ~1,587 cm −1 and ~2,647 cm −1 . However, some residual p-doping remains after the etching process. Patterning and electron transport of graphene nanoribbons We applied the DNA nanolithography technique to generate graphene nanoribbons. This allows us to test the method’s ability to generate extended structures with microns in length, commensurate in aspect ratio with a carbon nanotube. DNA ribbon templates with 60 nm width and several microns in length [26] were synthesized ( Fig. 4a ), and based on the same metallization-etching protocol, continuous graphene nanoribbons were fabricated all over the wafer surface. AFM ( Fig. 4b ) shows a graphene nanoribbon with an average height of 1.1±0.2 nm and up to ~10 μm in length. The width of the graphene nanoribbons matches that of the original DNA templates before metallization within the resolution limit of the AFM image [26] . Distribution in the width is expected from the observed curvature and curl of the DNA nanoribbons on the graphene surface and nonuniformity associated with the metallization process. 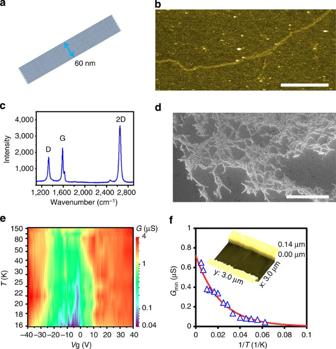Figure 4: Characterizations and electronic measurements of graphene nanoribbons. (a) Design of a SST DNA nanoribbon with 60 nm width, assembled by thousands of short-strand tiles. (b) AFM image of a graphene nanoribbon derived from metallized DNA nanolithography. Scale bar, 1 μm. (c) Raman spectrum of a single-layer graphene nanoribbon. (d) SEM image of graphene nanoribbons under an operation voltage of 1.0 kV. Scale bar, 10 μm. (e) The contour plot of the conductanceGof a graphene nanoribbon FET under different gate voltages and low temperatures. The appliedVdsis 0.1 V. (f) Minimum conductanceGminof a graphene nanoribbon device at different temperatures. The inset shows a 3D-rendered AFM topography of the device with a channel length of 2 μm. Figure 4: Characterizations and electronic measurements of graphene nanoribbons. ( a ) Design of a SST DNA nanoribbon with 60 nm width, assembled by thousands of short-strand tiles. ( b ) AFM image of a graphene nanoribbon derived from metallized DNA nanolithography. Scale bar, 1 μm. ( c ) Raman spectrum of a single-layer graphene nanoribbon. ( d ) SEM image of graphene nanoribbons under an operation voltage of 1.0 kV. Scale bar, 10 μm. ( e ) The contour plot of the conductance G of a graphene nanoribbon FET under different gate voltages and low temperatures. The applied V ds is 0.1 V. ( f ) Minimum conductance G min of a graphene nanoribbon device at different temperatures. The inset shows a 3D-rendered AFM topography of the device with a channel length of 2 μm. Full size image Raman spectroscopy suggests an average I D / I G value of ~0.7 for graphene nanoribbons ( Fig. 4c ), which is lower than those for letter-shaped graphene nanostructures ( I D / I G ~1.0) owing to the larger size. A high I D / I G value can be attributed to both bulk lattice defects [48] and atomically rough edges [53] , [57] . Because the perimeter-to-surface ratio is smaller for the wider graphene nanoribbons compared with the letter-shaped nanostructures, width confinement is diminished in the 60-nm wide ribbons, and we assign bulk defects to the graphene lattice accumulated throughout the different lithography steps, as the main contributors to the I D / I G value of the graphene nanoribbons. Unlike the letter-shaped graphene nanostructures that are hard to image with scanning electron microscopy (SEM) due to their tiny size and semiconductive nature, it is possible to observe the much longer graphene nanoribbons. A characteristic SEM image ( Fig. 4d ) shows that the graphene nanoribbons were distributed all over the substrate, highlighting the effectiveness for batch production of graphene ribbons via the metallized DNA masks. Field effect transistor (FET) devices based on the graphene nanoribbons were fabricated to characterize their electrical properties, as shown in Fig. 4e . Graphene nanoribbons were synthesized on a 300-nm thick SiO 2 /p-doped Si substrate, followed by EBL and deposition of Cr/Au to form source/drain contact electrodes on a target nanoribbon (see the inset of Fig. 4f ). The conductivity, G , of a 60-nm wide nanoribbon as a function of gate voltage, V g , was characterized at different temperatures T (16–200 K), as shown in Fig. 4e . The conductivity corresponding to high carrier density, n , does not vary over the temperature range considered; however, the minimum conductivity corresponding to n =0, G min , decreases significantly from 0.65 to 0.043 μS as the temperature decreases from 200 to 16 K. Therefore, the on/off current ratio increases approximately one order of magnitude from 200 to 16 K. The measured value of G min as a function of (1/ T ) is displayed in Fig. 4f . For the temperatures considered, we find that the conductivities are well described by the activation model with one activation energy, . The activation energy, E g , is approximately the transport band gap, indicating successful quantum confinement from the patterning [58] , [59] . For the device shown in Fig. 4f , the transport gap equals 3.9 meV, which is comparable to values obtained using EBL [6] or unzipping of carbon nanotubes [16] . This suggests that the defects and disorders generated during the metallization and etching processes do not increase carrier scattering compared with other methods. We conclude that this method is able to produce large amounts of micron-long graphene nanoribbons at wafer scale ( Fig. 4d ), with subsequent FET device qualities commensurated with previously published results obtained via other methods. The metallized DNA lithography does not disrupt Raman or electronic properties in the resulting products more than other methods do. Because it is possible to open a wider band gap by reducing the ribbon width [60] , the potential of programming ultra-narrow DNA templates is compelling and will be the subject of future efforts. In summary, we have demonstrated the first information transfer from encoded DNA nanostructures to another high-quality conductive material, such that metallized DNA templates can direct the formation of electronic devices. The cooperation between DNA self-assembly and 2D thin-film nanomaterials offers opportunities for both fields. Transferring structural information into graphene enables engineering of the electronic band diagram and quantum confinement of the resulting graphene nanostructures via the shape programmability of DNA nanostructures. Meanwhile self-assembled DNA structures expand the shape complexity of traditional lithographic processing for graphene, and this transfer allowed us to evaluate the imprinted fidelity for the first time using a convolution model. Prescribed 2D/3D DNA templates can be fabricated, enabling the production of not only linear, but also branched and ring-like graphene nanostructures. Scaling up the integration of graphene nanotransistors could be achieved through integrating circuit topology into larger size DNA masks that could be constructed using hierarchical or algorithmic self-assembly strategies. This would solve the difficulties of scaling up the fabrication of individual nanoscale graphene transistors with aligned orientation and location control. The DNA templates also make it possible to systematically alter the size of graphene nanostructures. A higher fabrication resolution will also be explored to enhance the quantum confinement and increase the transport gap of resulting FET devices. Another objective on this project is focusing on a unique, quantum interference transistor enabled by the patterned ring structures that we report in this paper. In addition to graphene, other atomic layered materials, such as MoS 2 and BN, may also be patterned with the current methodology for the design of diverse electronic devices. Preparation and transfer of monolayer CVD graphene Large-area monolayer graphene films were grown via CVD method on copper foils and then transferred to the surface of SiO 2 /Si wafers (with 300-nm thick thermally grown SiO 2 layer) [45] . Typically, an ~4 cm 2 copper foil (Aldrich, 99.999%, 25-μm thick) was placed at the centre of a 1-inch diameter fused quartz tube in a tube furnace. The furnace tube was evacuated and heated to 1,000 °C under a 30 sccm H 2 gas flow with a pressure of ~600 mTorr. After annealing for 30 min under these conditions, a CH 4 gas flow of 3.0 sccm was introduced and the temperature in the furnace tube was maintained at 1000 °C for 30 min. The CH 4 gas flow was stopped after the growth period. The copper foil was cooled to room temperature under H 2 gas flow and taken out from the tube furnace. A PMMA film was spin-coated (3,000 r.p.m., 1 min) onto the copper foil covered with CVD-graphene film and heated up to 150 °C for 2 min to cure the PMMA film. Then the PMMA/CVD-graphene layer was separated from the copper foil by etching in a 1 M CuCl 2 /6 M HCl aqueous solution and subsequently placed on the surface of Milli-Q water to remove any water-soluble residues. The PMMA/CVD-graphene film was then transferred to the designated substrate and dried with a nitrogen gun. The PMMA film was dissolved away by soaking the substrate in acetone for 6 h, thus leaving only the CVD-graphene sheet remaining on the substrate. Preparation of DNA nanorings DNA nanorings [24] were produced by mixing 100 nM of p7308 scaffold strand, 400 nM of each staple strand, purified by reverse-phase cartridge (Bioneer, Inc.), buffer and salts including 5 mM Tris (Fisher Scientific)+1 mM EDTA (Sigma-Aldrich, pH 8.0 at 20 °C) and 12 mM MgCl 2 (Fisher Scientific). The mixture was subjected to a thermal annealing ramp according to the following schedule: 80–61 °C at 5 min °C −1 , 60–24 °C at 150 min °C −1 . Crude products for DNA nanorings were purified by 2% native agarose gel electrophoresis (SYBR safe purchased from Invitrogen, freeze 'N Squeeze DNA gel extraction spin columns purchased from Bio-Rad, pellet pestles purchased from Scientific America and agarose purchased from Lonza). Preparation of letter-shaped DNA junctions Each specific shaped DNA letter [27] was produced by mixing 200 nM SST strands in 5 mM Tris+1 mM EDTA (pH 8.0 at 20 °C) and 12.5 mM MgCl 2 . The mixture was subjected to a thermal annealing ramp from 90 to 25 °C over 17 h according to the following schedule: 80–61 °C at 10 min °C −1 , 60–24 °C at 20 min °C −1 . Crude products for DNA letter-shapes were purified by 2% native agarose gel electrophoresis. Preparation of DNA nanoribbons DNA nanoribbons [26] were prepared by stoichiometrically mixing each SST strand to a final concentration of ~1 μM in 5 mM Tris+1 mM EDTA (pH 8.0 at 20 °C), and 12.5 mM MgCl 2 . The mixture was subjected to a thermal annealing ramp from 90 to 25 °C over 17 h according to the following schedule: 80–61 °C at 10 min °C −1 , 60–24 °C at 20 min °C −1 . Glutaraldehyde treatment of DNA nanostructures Purified self-assembled DNA nanostructures were incubated with 0.2% glutaraldehyde (Sigma-Aldrich) diluted in 0.5 × TBE/10 mM MgCl 2 buffer on ice for 20 min and then at room temperature for another 20 min, after which the sample was loaded into a spin column with Molecular Weight Cut Off (MWCO) of 100 kDa (Millipore) and washed with 500 μl 0.5 × TBE/10 mM MgCl 2 for three times to remove the excess glutaraldehyde. Deposition of DNA nanostructures on graphene To get better affinity with negatively charged DNA structures, graphene samples were firstly dipped into 0.1 mg ml −1 1-pyrenemethylamine methanol solution for 5 min, and then gently dried with a nitrogen gun. We also tried 1-pyrenebutylcarboxylic acid, 1-pyrenesulfonate and 4-(1-Pyrene) butyric acid N-hydroxysuccinimide ester as controls. We found that among these chemicals, 1-pyrenemethylamine provides the best dispersion of DNA on the surface of graphene. Subsequently, 5 μl of glutaraldehyde-treated DNA in 0.5 × TBE/10 mM MgCl 2 buffer was dropped onto graphene surface. Five minutes later, when the DNA drop had nearly completely dried in air, the graphene sample was rinsed in water twice for 15 s to remove excessive glutaraldehyde and residual buffer, and then dried with a nitrogen gun. DNA metallization The graphene sample covered with glutaraldehyde-treated DNA was incubated in the dark with a 0.1 M solution of AgNO 3 in ammonia buffer (pH=10.5) at room temperature for 1 h to trigger the growth of silver seeds on DNA skeletons, after which the excessive reagents were rinsed off with deionized water. Final incubation with Gold Enhance EM Formulation (Nanoprobes) was processed according to the manufacturer’s instructions. First, a unit of enhancer (A) was mixed with a unit of activator (B), and then a unit of initiator (C) and a unit of buffer (D) was added to the mixture. A volume of 10 μl of this mixture was freshly deposited onto a graphene substrate and incubated for 2 min to produce gold-covered DNA nanostructures. Excess reagent was rinsed off form the sample with deionized water. Etching of graphene nanostructures The graphene samples covered with metallized DNA masks were exposed to RIE conditions (10 mTorr Ar and 10 mTorr O 2 flow at 50 W for 8 s in a Nexx ECR RIE system) to remove the unprotected region of graphene. Mask removal The RIE-treated samples were soaked in 0.1 M NaCN/H 2 O solution for 10 min to remove metal masks, and then rinsed in water for 10 s. Subsequently, the samples were put into 99.5% deionized formamide for another 10 min and then rinsed in water for 10 s to remove any possible DNA residue. Characterizations and electronic measurements AFM was conducted on an Asylum Research MFP-3D system in AC mode (alternating current mode, also called noncontact or tapping mode) using silicon probes (Olympus OMCL-AC240TS). Raman spectroscopy was performed on a Horiba Jobin Yvon LabRAM HR800 system using a 633-nm excitation laser, × 100 objective lens with ~1 μm diameter spot size and 600 lines per mm grating. All the Raman spectra were collected with exposure time of 5 s and accumulated two times. The Raman peaks are fit to Lorentzians after background subtraction. SEM was performed on a Zeiss FESEM Ultra Plus system under high vacuum and operation voltage of 1 kV. Back-gated graphene nanoribbon devices on 300 nm SiO 2 /Si substrates were fabricated using conventional lithography and the source/drain electrodes were prepared by electron beam deposition of 25/75-nm thick Cr/Au layers sequentially under high vacuum. Electronic measurements of the graphene nanoribbon FET devices were collected with an ARS PSF-10-1-4 Cryogenic Probe Station and an Agilent E5270B analyzer at 15–200 K and pressure <10 −6 Torr. How to cite this article: Jin, Z. et al . Metallized DNA nanolithography for encoding and transferring spatial information for graphene patterning. Nat. Commun. 4:1663 doi: 10.1038/ncomms2690 (2013).